Peptide hormone ghrelin enhances neuronal excitability by inhibition of Kv7/KCNQ channels The gut-derived orexigenic peptide hormone ghrelin enhances neuronal firing in the substantia nigra pars compacta, where dopaminergic neurons modulate the function of the nigrostriatal system for motor coordination. Here we describe a novel mechanism by which ghrelin enhances firing of nigral dopaminergic neurons by inhibiting voltage-gated potassium Kv7/KCNQ/M-channels through its receptor GHS-R1a and activation of the PLC-PKC pathway. Brain slice recordings of substantia nigra pars compacta neurons reveal that ghrelin inhibits native Kv7/KCNQ/M-currents. This effect is abolished by selective inhibitors of GHS-R1a, PLC and PKC. Transgenic suppression of native Kv7/KCNQ/M-channels in mice or channel blockade with XE991 abolishes ghrelin-induced hyperexcitability. In vivo , intracerebroventricular ghrelin administration causes increased dopamine release and turnover in the striatum. Microinjection of ghrelin or XE991 into substantia nigra pars compacta results in contralateral dystonic posturing, and attenuation of catalepsy elicited by systemic administration of the D2 receptor antagonist haloperidol. Our findings indicate that the ghrelin/KCNQ signalling is likely a common pathway utilized by the nervous system. The excitability of dopaminergic neurons in the substantia nigra pars compacta (SNc) that supply the striatum with dopamine determines the function of nigrostriatal system for motor coordination [1] . Dysfunction of dopaminergic neurotransmission has been implicated in a variety of neuropsychiatric disorders [2] , [3] . Parkinson’s disease (PD) is a progressive neurodegenerative disorder characterized by the loss of dopaminergic neurons in SNc with major symptoms including resting tremor, akynesia and disturbance of posture [4] . One practical approach for alleviation of PD symptoms is to enhance the excitability of surviving dopaminergic neurons in SNc where the neuronal activity can be modulated by a variety of neurotransmitters, endogenous hormones and peptides [5] , [6] . Ghrelin, an endogenous ligand for growth hormone secretagogue receptor (GHS-R, a G-protein-coupled receptor), is a 28-amino-acid peptide that regulates growth hormone secretion, food intake, reward-seeking behaviour and memory performance [7] , [8] , [9] , [10] . It is mainly secreted from stomach [7] , with small amounts produced in the brain [11] . GHS-R is expressed in various brain areas including SNc, hypothalamus, ventral tegmental area and hippocampus where ghrelin directly modulates the neuronal activity [9] , [10] , [12] , [13] . In SNc, ghrelin electrically activates dopaminergic neurons, and increases dopamine concentration in the striatum [12] . However, how ghrelin enhances neuronal excitability remains largely unknown. Neuronal M-current is a subthreshold voltage-gated K + current encoded by Kv7/KCNQ channels that modulate firing frequency of mesencephalic dopamine neurons [14] and are functionally coupled to dopamine D2 receptors, providing essential modulatory inputs to their striatal and limbic targets [15] , [16] . Both Kv7/KCNQ channels and GHS-R are expressed in the SNc, hippocampus, dorsal root ganglion (DRG), hypothalamus and cortex [11] , [15] , [17] , [18] , [19] , [20] , [21] , [22] , [23] . KCNQ channels are also negatively modulated by G-protein-coupled receptors via Gq and/or G 11 activated phospholipase C (PLC)-mediated signal pathway [24] , [25] , [26] . It has also been reported that the effects of ghrelin are mediated by PLC that hydrolyses PIP 2 for IP 3 signalling in hypothalamus [13] , or by protein kinase C (PKC) in non-neuronal tissues and cell lines [27] , [28] , ultimately affecting potassium channel conductance [29] . All these observations suggest that ghrelin signalling is likely coupled with neuronal KCNQ/M-channel function. In this study, we sought to understand the molecular mechanism and signalling pathway of how ghrelin regulates the excitability of nigral dopaminergic neurons. Here, we show that central ghrelin enhances dopaminergic neuronal excitability by inhibiting Kv7/KCNQ/M-channel via the GHS-R1a-PLC-PKC pathway in vitro , and improves motor coordination in vivo . Ghrelin enhances excitability of dopaminergic neurons in SNc We started by examining effects of ghrelin on electrical properties of nigral dopaminergic neurons from rat brain slices. Dopaminergic neurons in SNc were identified by the following criteria: (i) Medium-to-large cell body with triangular or fusiform shapes in diameter about 20.1±0.9 μm ( Fig. 1a , left panel); (ii) presence of a large sag in response to hyperpolarizing current injection and regular firing in response to small current injections ( Fig. 1a , middle panel); (iii) broad action potential with half width of 3.2±0.1 ms ( Fig. 1a , right panel); (iv) low-frequency pacemaker activity about 1.2±0.1 Hz ( Fig. 1b , left panel). 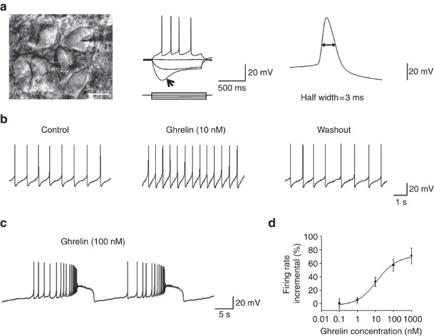Figure 1: Ghrelin increases excitability of dopaminergic neurons in substantia nigra. (a) Dentification of dopaminergic neurons in SNc. Left panel shows recording of a putative dopaminergic neuron characterized by large cell body (26 μm) and triangular multipolar shape under Differential Interference Contrast microscope. Middle panel: dopaminergic neurons were further identified by the presence of a large sag (arrow) in the voltage response to hyperpolarizing current steps. The example neuron fired regular spikes in response to 50 pA injection. Below shows the current steps from −100 pA with 50-pA increments. Right panel: the expanded view of an action potential showing the half width of 3 ms. (b) Representative raw traces of spontaneous action potentials were recorded before, during, and after application of ghrelin (10 nM,n=43). A concentration of 10 nM ghrelin reversibly increased the firing frequency from 1.2 Hz to 1.5 Hz for the example neuron. (c) High concentration of ghrelin (100 nM) changed the neuronal discharge pattern from pacemaker mode to burst firing. (d) Dose–response curve for ghrelin in which firing rate is plotted against ghrelin concentrations from 0.1 to 1,000 nM (n=6–9). Data were fitted to a sigmoid dose–response function with half maximal effective concentration (EC50) of 12.3 nM. Each bar represents the mean±s.e.m. Scale bar, (left), 20 μm (a). Figure 1: Ghrelin increases excitability of dopaminergic neurons in substantia nigra. ( a ) Dentification of dopaminergic neurons in SNc. Left panel shows recording of a putative dopaminergic neuron characterized by large cell body (26 μm) and triangular multipolar shape under Differential Interference Contrast microscope. Middle panel: dopaminergic neurons were further identified by the presence of a large sag (arrow) in the voltage response to hyperpolarizing current steps. The example neuron fired regular spikes in response to 50 pA injection. Below shows the current steps from −100 pA with 50-pA increments. Right panel: the expanded view of an action potential showing the half width of 3 ms. ( b ) Representative raw traces of spontaneous action potentials were recorded before, during, and after application of ghrelin (10 nM, n =43). A concentration of 10 nM ghrelin reversibly increased the firing frequency from 1.2 Hz to 1.5 Hz for the example neuron. ( c ) High concentration of ghrelin (100 nM) changed the neuronal discharge pattern from pacemaker mode to burst firing. ( d ) Dose–response curve for ghrelin in which firing rate is plotted against ghrelin concentrations from 0.1 to 1,000 nM ( n =6–9). Data were fitted to a sigmoid dose–response function with half maximal effective concentration (EC 50 ) of 12.3 nM. Each bar represents the mean±s.e.m. Scale bar, (left), 20 μm ( a ). Full size image To investigate the effect of ghrelin on spontaneous firing of nigral dopaminergic neurons, we applied ghrelin to the bath. Ghrelin at low concentration (10 nM) significantly increased the firing rate, and the effect could be washed out ( Fig. 1b ). Increasing ghrelin concentrations (100 nM) resulted in bursting firing ( Fig. 1c ) and a dose-dependent increase in firing rate with an half maximal effective concentration (EC 50 ) of 12.3 nM ( n =6–9) ( Fig. 1d ). Previous studies indicated that ghrelin might enhance dopaminergic neuronal excitability through modulating synaptic activity in ventral tegmental area [9] . To exclude this possibility in SNc, we added both excitatory and inhibitory synaptic inhibitors (20 μM CNQX, 50 μM AP5 and 10 μM bicuculline) in the recording solution. Ghrelin (10 nM) increased the neuronal firing rate either under whole-cell configuration or perforated patch clamp recordings ( Supplementary Fig. S1 ), suggesting that ghrelin might directly activate nigral dopaminergic neurons. To examine whether the increased excitability of dopaminergic neurons by ghrelin was mediated through activation of its receptor GHS-R1a (a G-protein-coupled receptor), a receptor-selective peptide antagonist, D -[Lys3]-GHRP-6, was applied before the administration of ghrelin. As shown in Fig. 2a , bath application of D -[Lys3]-GHRP-6 (50 μM) alone had no effect on firing. In contrast, when added together with ghrelin, D -[Lys3]-GHRP-6 completely abolished the ghrelin-induced increase of firing. This result suggests that the effect of ghrelin is mediated by activating its receptor GHS-R1a. 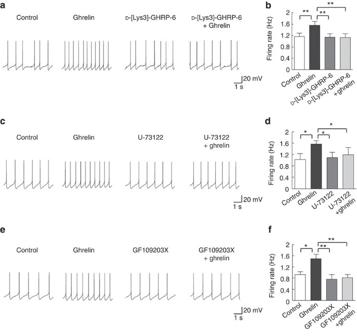Figure 2: Ghrelin increases spontaneous firing of dopaminergic neurons via the GHS-R1a-PLC-PKC pathway. (a) Raw traces show the spontaneous firing in the absence or presence of ghrelin and GHS-R1a antagonistD-[Lys3]-GHRP-6. Ghrelin (10 nM) increased firing frequency andD-[Lys3]-GHRP-6 (50 μM) alone had no effect on neuronal firing. Co-application ofD-[Lys3]-GHRP-6 and ghrelin abolished stimulatory effect of ghrelin on neuronal firing. (b) A summary of statistical analysis for firing frequency froma(n=7). Each bar represents the mean±s.e.m. **P<0.01, Ghrelin versus Control; **P<0.01, Ghrelin versusD-[Lys3]-GHRP-6; **P<0.01, Ghrelin versus (D-[Lys3]-GHRP-6 + Ghrelin);F=4.950, analysis of variance (ANOVA) followed by Student-Newman-Keuls (S-N-K) test. (c–f) Summary of effects of inhibitors on ghrelin signalling transduction pathways. Both PLC inhibitor U-73122 and PKC inhibitor GF109203X diminished ghrelin effect. (c) PLC inhibitor U-73122 (10 μM) alone had no effect on neuronal firing, co-application of U-73122 (10 μM) and ghrelin (10 nM) abolished stimulatory effect of ghrelin on neuronal firing. (d) A summary of statistical analysis for firing frequency fromc(n=7). Each bar represents the mean±s.e.m. *P<0.05, Ghrelin versus Control; *P<0.05, Ghrelin versus U-73122; *P<0.05, Ghrelin versus (U-73122 + Ghrelin);F=3.9, ANOVA followed by S-N-K test. (e) PKC inhibitor GF109203X (5 μM) alone had no effect on neuronal firing, co-application of GF109203X (5 μM) and ghrelin (10 nM) abolished stimulatory effect of ghrelin on neuronal firing. (f) A summary of statistical analysis for firing frequency frome(n=9). Each bar represents the mean±s.e.m. *P<0.05, Ghrelin versus Control; **P<0.01, Ghrelin versus GF109203X; **P<0.01, Ghrelin versus (GF109203X + Ghrelin);F=5.807, ANOVA followed by S-N-K test. Figure 2: Ghrelin increases spontaneous firing of dopaminergic neurons via the GHS-R1a-PLC-PKC pathway. ( a ) Raw traces show the spontaneous firing in the absence or presence of ghrelin and GHS-R1a antagonist D -[Lys3]-GHRP-6. Ghrelin (10 nM) increased firing frequency and D -[Lys3]-GHRP-6 (50 μM) alone had no effect on neuronal firing. Co-application of D -[Lys3]-GHRP-6 and ghrelin abolished stimulatory effect of ghrelin on neuronal firing. ( b ) A summary of statistical analysis for firing frequency from a ( n =7). Each bar represents the mean±s.e.m. ** P <0.01, Ghrelin versus Control; ** P <0.01, Ghrelin versus D -[Lys3]-GHRP-6; ** P <0.01, Ghrelin versus ( D -[Lys3]-GHRP-6 + Ghrelin); F =4.950, analysis of variance (ANOVA) followed by Student-Newman-Keuls (S-N-K) test. ( c – f ) Summary of effects of inhibitors on ghrelin signalling transduction pathways. Both PLC inhibitor U-73122 and PKC inhibitor GF109203X diminished ghrelin effect. ( c ) PLC inhibitor U-73122 (10 μM) alone had no effect on neuronal firing, co-application of U-73122 (10 μM) and ghrelin (10 nM) abolished stimulatory effect of ghrelin on neuronal firing. ( d ) A summary of statistical analysis for firing frequency from c ( n =7). Each bar represents the mean±s.e.m. * P <0.05, Ghrelin versus Control; * P <0.05, Ghrelin versus U-73122; * P <0.05, Ghrelin versus (U-73122 + Ghrelin); F =3.9, ANOVA followed by S-N-K test. ( e ) PKC inhibitor GF109203X (5 μM) alone had no effect on neuronal firing, co-application of GF109203X (5 μM) and ghrelin (10 nM) abolished stimulatory effect of ghrelin on neuronal firing. ( f ) A summary of statistical analysis for firing frequency from e ( n =9). Each bar represents the mean±s.e.m. * P <0.05, Ghrelin versus Control; ** P <0.01, Ghrelin versus GF109203X; ** P <0.01, Ghrelin versus (GF109203X + Ghrelin); F =5.807, ANOVA followed by S-N-K test. Full size image Since GHS-R1a is a G-protein-coupled PLC-dependent receptor, we next tested whether ghrelin’s effect was mediated by activation of GHS-R1a downstream signalling pathway. As a control, application of either a selective PLC inhibitor U-73122 (10 μM) ( Fig. 2c ) or PKC inhibitor GF109203X (5 μM) ( Fig. 2e ) alone had no effect on firing rate. In contrast, either U-73122 (10 μM) or GF109203X (5 μM) abolished ghrelin-induced effect on firing rate ( Fig. 2c–f ). These results demonstrate that the GHS-R1a-PLC-PKC pathway is involved in the effects of ghrelin on dopaminergic neurons in SNc. Inhibition of voltage-dependent KCNQ/M-currents by ghrelin To test the effect of ghrelin on neuronal KCNQ/M-current in SNc, we first performed nystatin-perforated patch clamp recordings of brain slices and characterized the native current in the presence of KCNQ channel specific blocker XE991. KCNQ/M-currents in the nigral dopaminergic neurons were examined using a standard deactivation protocol [17] , [22] , [30] . Neurons were constantly held at −20 mV to minimize contamination from currents such as A-type potassium current or sodium current. KCNQ-like currents could be visualized with a 1-s-long hyperpolarizing voltage steps from −20 mV to −30~−40 mV. When holding potential was stepped to −30 from −20 mV, a typical deactivation relaxation of KCNQ/M-current was observed ( Fig. 3a , left panel), and time-dependent activation current was also easily seen when holding potential stepped back to −20 mV ( Fig. 3a , left panel). The deactivation time constant was about 185±18.3 ms at −40 mV, which is comparable to that of KCNQ current recorded in dopaminergic neurons of ventral tegmental area [22] . The amplitude of KCNQ current in SNc was 20.9±7.4 pA when measured at −40 mV ( n =13, Fig. 3c ). Addition of KCNQ/M-channel-specific blocker XE991 (30 μM) strongly inhibited this current from 24.3±7.5 to 5.5±2.1 pA ( Fig. 3a ), and the isolated XE991-sensitive current shared the similar properties with typical native KCNQ/M-current ( Fig. 3b ). 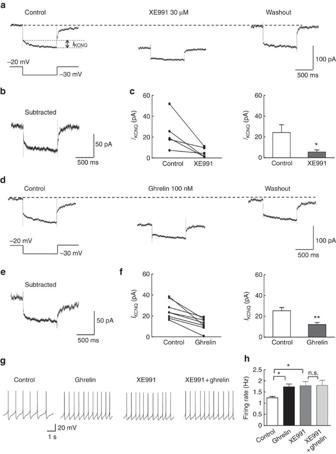Figure 3: Ghrelin inhibits KCNQ current in nigral dopaminergic neurons. (a) Characterizations of KCNQ currents in SNc neurons by nystatin-perforated patch clamp recording using the standard deactivation protocol. KCNQ current showed characteristic inward relaxation when recorded from the holding potential of −20 to −30 mV and the time-dependent activation when stepped back to −20 mV. Dashed line indicates the current measured at −20 mV before the application of XE991. XE991 (30 μM) diminished the inward relaxation current caused by deactivation and elicited obvious baseline drops at −20 mV, reflecting the closure of KCNQ channels. (b) The enlarged subtracted trace of XE991-sensitive current calculated froma. (c) Left panel: the amplitude of KCNQ currents (IKCNQ) quantified from all SNc neurons held at −20 to −40 mV in the presence or absence of XE991. Right panel:IKCNQwas inhibited by 30 μM XE991 (n=5. Each bar represents the mean±s.e.m. *P<0.05, XE991 versus Control,t=2.186, Pairedt-test.). (d) KCNQ currents recorded before, during and after application of ghrelin (100 nM,n=12). Ghrelin inhibited the KCNQ current in a reversible manner. (e) The enlarged subtracted trace of ghrelin-sensitive current (calculated fromd) possesses the deactivation relaxation and activation kinetics of KCNQ current. (f) Left panel:IKCNQquantified from all neurons recorded from a holding potential of −20 to −40 mV in the presence or absence of ghrelin. Right panel shows the statistical analysis of data from the left panel.IKCNQwas inhibited in the presence of 100 nM ghrelin (n=8. Each bar represents the mean±s.e.m. **P<0.01, Ghrelin versus Control,t=5.206, Pairedt-test.). (g) XE991 abolished the excitatory effect of ghrelin. Both ghrelin and XE991 increased the firing rate. However, ghrelin (10 nM) failed to further increase firing rate in the presence of XE991 (1 μM). (h) A summary of statistical analysis forg.n=8. Each bar represents the mean±s.e.m. *P<0.05, Ghrelin versus Control; *P<0.05, XE991 versus Control; n.s., no significant difference, XE991 versus (XE991 + Ghrelin);F=3.452, ANOVA followed by S-N-K test. Figure 3: Ghrelin inhibits KCNQ current in nigral dopaminergic neurons. ( a ) Characterizations of KCNQ currents in SNc neurons by nystatin-perforated patch clamp recording using the standard deactivation protocol. KCNQ current showed characteristic inward relaxation when recorded from the holding potential of −20 to −30 mV and the time-dependent activation when stepped back to −20 mV. Dashed line indicates the current measured at −20 mV before the application of XE991. XE991 (30 μM) diminished the inward relaxation current caused by deactivation and elicited obvious baseline drops at −20 mV, reflecting the closure of KCNQ channels. ( b ) The enlarged subtracted trace of XE991-sensitive current calculated from a . ( c ) Left panel: the amplitude of KCNQ currents ( I KCNQ ) quantified from all SNc neurons held at −20 to −40 mV in the presence or absence of XE991. Right panel: I KCNQ was inhibited by 30 μM XE991 ( n =5. Each bar represents the mean±s.e.m. * P <0.05, XE991 versus Control, t =2.186, Paired t -test.). ( d ) KCNQ currents recorded before, during and after application of ghrelin (100 nM, n =12). Ghrelin inhibited the KCNQ current in a reversible manner. ( e ) The enlarged subtracted trace of ghrelin-sensitive current (calculated from d ) possesses the deactivation relaxation and activation kinetics of KCNQ current. ( f ) Left panel: I KCNQ quantified from all neurons recorded from a holding potential of −20 to −40 mV in the presence or absence of ghrelin. Right panel shows the statistical analysis of data from the left panel. I KCNQ was inhibited in the presence of 100 nM ghrelin ( n =8. Each bar represents the mean±s.e.m. ** P <0.01, Ghrelin versus Control, t =5.206, Paired t -test.). ( g ) XE991 abolished the excitatory effect of ghrelin. Both ghrelin and XE991 increased the firing rate. However, ghrelin (10 nM) failed to further increase firing rate in the presence of XE991 (1 μM). ( h ) A summary of statistical analysis for g . n =8. Each bar represents the mean±s.e.m. * P <0.05, Ghrelin versus Control; * P <0.05, XE991 versus Control; n.s., no significant difference, XE991 versus (XE991 + Ghrelin); F =3.452, ANOVA followed by S-N-K test. Full size image Application of ghrelin (100 nM) in the presence or absence of synaptic blockers resulted in the inhibition of KCNQ/M-current recorded under the standard deactivation protocol (12 out of 14 neurons) from 25.4±3 to 12.1±2.1 pA ( Figs 3d and 4a ). Further analysis of ghrelin-sensitive current, subtracted by ghrelin-resistant current from the original trace, revealed that ghrelin-inhibited current is primarily KCNQ/M-current ( Fig. 3e ). The remaining ghrelin-resistant neurons were also not responsive to XE991, possibly due to the lack of KCNQ expression in those neurons. The specific channel blocker XE991 (1 μM) significantly enhanced the spontaneous firing of dopaminergic neurons, whereas further application of ghrelin (10 nM) had no additional effect on neuronal firing ( Fig. 3g ). 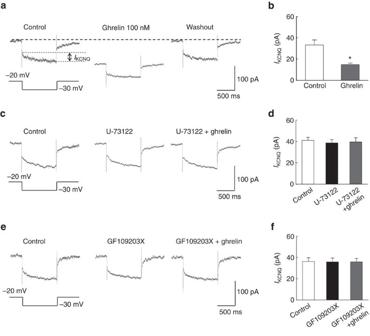Figure 4: Ghrelin inhibits KCNQ current in nigral dopaminergic neurons via PLC and PKC. The SNc dopaminergic neurons were recorded under perforated patch clamp recordings in the presence of synaptic blockers (20 μM CNQX+50 μM AP5+10 μM bicuculline). (a) Ghrelin (100 nM) inhibited KCNQ currents in the presence of synaptic blockers. (b) Statistical analysis fora.n=3. Each bar represents the mean±s.e.m. *P<0.05, Ghrelin versus Control,t=5.526, Pairedt-test. (c) Representative data showed that PLC inhibitor U-73122 (10 μM) alone had no effect on KCNQ current, however, it could abolish ghrelin’s effects on KCNQ current inhibition. (d) Statistical analysis forc.n=3. Each bar represents the mean±s.e.m. (e) PKC inhibitor GF109203X (5 μM) abolished the inhibitory effects of ghrelin on KCNQ current. (f) Statistical analysis fore.n=3. Each bar represents the mean±s.e.m. Figure 4: Ghrelin inhibits KCNQ current in nigral dopaminergic neurons via PLC and PKC. The SNc dopaminergic neurons were recorded under perforated patch clamp recordings in the presence of synaptic blockers (20 μM CNQX+50 μM AP5+10 μM bicuculline). ( a ) Ghrelin (100 nM) inhibited KCNQ currents in the presence of synaptic blockers. ( b ) Statistical analysis for a . n =3. Each bar represents the mean±s.e.m. * P <0.05, Ghrelin versus Control, t =5.526, Paired t -test. ( c ) Representative data showed that PLC inhibitor U-73122 (10 μM) alone had no effect on KCNQ current, however, it could abolish ghrelin’s effects on KCNQ current inhibition. ( d ) Statistical analysis for c . n =3. Each bar represents the mean±s.e.m. ( e ) PKC inhibitor GF109203X (5 μM) abolished the inhibitory effects of ghrelin on KCNQ current. ( f ) Statistical analysis for e . n =3. Each bar represents the mean±s.e.m. Full size image As GHS-R1a-PLC-PKC pathway is involved in the effect of ghrelin on neuronal firing, we further investigated whether PLC and PKC are necessary for the inhibition of KCNQ/M-current by ghrelin. Both U-73122 (10 μM) and GF109203X (5 μM) prevented ghrelin from inhibiting KCNQ/M-current ( Fig. 4c–f ). These results demonstrate that ghrelin enhances dopaminergic neuronal firing by inhibiting KCNQ/M-current through PLC-PKC signalling pathway. KCNQ channel block diminishes the effects of ghrelin To make sure that excitatory effect of ghrelin was indeed mediated through the inhibition of native KCNQ/M-current, we took advantage of the robust expression of KCNQ current in DRG neurons (at least 50 times larger than that recorded in SNc) [17] . To recapitulate the observation in SNc, we first tested the effect of ghrelin on firing rate of DRG neurons (with capacitance 21.6±1.6 pF, ranging from 14 to 34 pF, Fig. 5b ). DRG neurons are highly refractory [17] , and typically fired at 1–2 spikes in response to 200~250 pA current injection ( Fig. 5a ). Administration of ghrelin (300 nM) increased the number of spikes under the same condition, and this effect could be slowly washed out in more than 20 min ( Fig. 5a ). Similar to the effect of ghrelin on firing rate in SNc, XE991 (30 μM) increased the firing rate ( Fig. 5c ), and addition of ghrelin (300 nM) in the presence of XE991 had no effect on further increase of firing, suggesting that blocking native KCNQ current can prevent ghrelin from further inhibition of KCNQ/M-current. 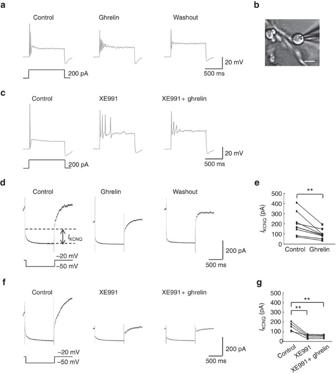Figure 5: KCNQ-specific blocker XE991 abolishes ghrelin’s effect on DRG neurons. (a) Ghrelin increased evoked firing of DRG neurons. The evoked action potentials were shown before (control), during (ghrelin) and after (washout) application of 300 nM ghrelin in the bath (n=7). One or two spikes were produced by a 200-pA depolarizing current pulse in the control, whereas multiple spikes were produced in response to the same current injection in the presence of 300 nM ghrelin. (b) Recording of a cultured DRG neuron under Differential Interference Contrast microscope. Scale bar, 20 μm. (c) XE991 (30 μM,n=5) increased the evoked neuronal firing (left and middle panel). Ghrelin (300 nM,n=5) failed to further increase the evoked neuronal firing in the presence of 30 μM XE991 (right panel). (d) KCNQ currents were recorded before (control), during (ghrelin) and after (washout) application of 300 nM ghrelin using the standard deactivation protocol from −20 to −50 mV. Ghrelin significantly inhibited the KCNQ current (n=9), and the response could be washout (n=5). (e) Statistical analysis of KCNQ currents quantified from all DRG neurons held at −20 to −50 mV in the presence or absence of ghrelin (n=5). The KCNQ current of all DRG neurons were significantly inhibited by 300 nM ghrelin (n=9, **P<0.01, Ghrelin versus Control;t=4.094, Pairedt-test). (f) KCNQ current was almost abolished by prolonged application of 30 μM XE991, further application of ghrelin (300 nM) had no effect on residual current. (g) Statistical analysis off(n=5, **P<0.01, XE991 versus Control; **P<0.01, (XE991+Ghrelin) versus Control;F=19.058, analysis of variance followed by S-N-K test). Figure 5: KCNQ-specific blocker XE991 abolishes ghrelin’s effect on DRG neurons. ( a ) Ghrelin increased evoked firing of DRG neurons. The evoked action potentials were shown before (control), during (ghrelin) and after (washout) application of 300 nM ghrelin in the bath ( n =7). One or two spikes were produced by a 200-pA depolarizing current pulse in the control, whereas multiple spikes were produced in response to the same current injection in the presence of 300 nM ghrelin. ( b ) Recording of a cultured DRG neuron under Differential Interference Contrast microscope. Scale bar, 20 μm. ( c ) XE991 (30 μM, n =5) increased the evoked neuronal firing (left and middle panel). Ghrelin (300 nM, n =5) failed to further increase the evoked neuronal firing in the presence of 30 μM XE991 (right panel). ( d ) KCNQ currents were recorded before (control), during (ghrelin) and after (washout) application of 300 nM ghrelin using the standard deactivation protocol from −20 to −50 mV. Ghrelin significantly inhibited the KCNQ current ( n =9), and the response could be washout ( n =5). ( e ) Statistical analysis of KCNQ currents quantified from all DRG neurons held at −20 to −50 mV in the presence or absence of ghrelin ( n =5). The KCNQ current of all DRG neurons were significantly inhibited by 300 nM ghrelin ( n =9, ** P <0.01, Ghrelin versus Control; t =4.094, Paired t -test). ( f ) KCNQ current was almost abolished by prolonged application of 30 μM XE991, further application of ghrelin (300 nM) had no effect on residual current. ( g ) Statistical analysis of f ( n =5, ** P <0.01, XE991 versus Control; ** P <0.01, (XE991+Ghrelin) versus Control; F =19.058, analysis of variance followed by S-N-K test). Full size image We further examined the direct effect of ghrelin on native KCNQ/M-current recorded from DRG neurons. As shown in Fig. 5d , standard deactivation protocol elicited the typical KCNQ/M-current, and the addition of ghrelin (300 nM) inhibited the KCNQ/M-current significantly from 197.9±36.2 pA to 98.3±16 pA, and this effect could be washed out. In the presence of XE991, further application of ghrelin had little effect on KCNQ/M-current ( Fig. 5f ), consistent with the results obtained from ghrelin on firing ( Fig. 5c ). Suppression of KCNQ function diminishes ghrelin effects To further confirm the role of ghrelin/KCNQ pathway in neuronal excitability, we utilized transgenic (Tg) mice carrying a dominant negative pore mutation of Kv7.2/KCNQ2 channel (rQ2-G279S) under the control of forebrain-specific aCaMKII promoter [31] . While CA1 pyramidal neurons from WT mice express typical KCNQ/M-current, the KCNQ/M-current of Tg mice was significantly suppressed ( Fig. 6a ). CA1 pyramidal neurons in WT mice fired spontaneously at low frequency under perforated patch clamp ( Fig. 6c ), and ghrelin (100 nM) increased the firing rate from 1.5±0.4 Hz to 2.1±0.4 Hz ( n =8, P <0.01, Fig. 6c ). Compared with WT mice, the spontaneous firing rate of Tg mice increased to 2.7±0.4 Hz, whereas ghrelin failed to further increase the firing rate (2.8±0.4 Hz, n =11) ( Fig. 6e ). It is noted that the KCNQ/M-currents are not totally suppressed in all neurons recorded. Considering the individual neurons of Tg mice, 8 out of 11 neurons did not respond to ghrelin, the remaining 3 neurons bearing normal KCNQ/M-current indeed increased firing rate, further demonstrating the necessity of KCNQ channel in promoting neuronal firing by ghrelin. When considered at population level, as shown in Fig. 6g , ghrelin (100 nM) significantly increased the firing rate of WT neurons, and in contrast, neurons from Tg mice showed no further increase in the presence of same concentration of ghrelin. These results demonstrated that ghrelin could not further increase the firing rate of CA1 pyramidal neurons where KCNQ/M-current was inhibited, indicating the role of ghrelin/KCNQ pathway in controlling neuronal excitability. Loss of sensitivity to ghrelin of CA1 pyramidal neurons of Tg mice seems not due to the lack of expression of ghrelin receptor, because the expression pattern of GHS-R1a in CA1 of Tg mice was similar to that of WT mice ( Supplementary Fig. S2 ). Taken together, all these results indicate that ghrelin functions as an upstream signalling molecule and ghrelin-KCNQ pathway is commonly shared in neurons from hippocampus, SNc and DRG. 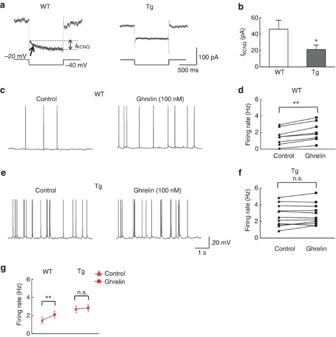Figure 6: Attenuation of ghrelin-mediated enhancement of firing in CA1 pyramidal neurons from Tg mice. (a) KCNQ currents of example CA1 pyramidal neurons in wild type (WT) and Tg mice recorded by nystatin-perforated patch clamp recording under standard deactivation protocol from the holding potential of −20 to −40 mV. Note the pronounced deactivation relaxation (arrow in left panel) of WT mice, which was absence in the example neuron of Tg mice. (b) Statistical analysis of amplitude of native KCNQ current (IKCNQ) in WT (n=7) and Tg (n=11) mice (each bar represents the mean±s.e.m. *P<0.05, WT versus Tg;t=2.279, unpairedt-test.). (c) The example CA1 pyramidal neuron of WT mice fired spontaneous action potential at 0.6 Hz. A concentration of 100 nM ghrelin significantly increased firing rate to 1.2 Hz. (d) Collective data of all neurons recorded. Ghrelin increased the firing rate of all neurons (8/8) in WT mice (**P<0.01, Ghrelin versus Control,t=7.570, Pairedt-test). (e) Raw traces showing that ghrelin did not change the firing rate of the example neuron in Tg mice. (f) In Tg mice, the firing rate of neurons (8/11) was not increased in the presence of 100 nM ghrelin (n.s. ghrelin versus control,t=1.112, Pairedt-test). (g) Statistical analysis ofdandf. Each bar represents the mean±s.e.m. Figure 6: Attenuation of ghrelin-mediated enhancement of firing in CA1 pyramidal neurons from Tg mice. ( a ) KCNQ currents of example CA1 pyramidal neurons in wild type (WT) and Tg mice recorded by nystatin-perforated patch clamp recording under standard deactivation protocol from the holding potential of −20 to −40 mV. Note the pronounced deactivation relaxation (arrow in left panel) of WT mice, which was absence in the example neuron of Tg mice. ( b ) Statistical analysis of amplitude of native KCNQ current ( I KCNQ ) in WT ( n =7) and Tg ( n =11) mice (each bar represents the mean±s.e.m. * P <0.05, WT versus Tg; t =2.279, unpaired t -test.). ( c ) The example CA1 pyramidal neuron of WT mice fired spontaneous action potential at 0.6 Hz. A concentration of 100 nM ghrelin significantly increased firing rate to 1.2 Hz. ( d ) Collective data of all neurons recorded. Ghrelin increased the firing rate of all neurons (8/8) in WT mice (** P <0.01, Ghrelin versus Control, t =7.570, Paired t -test). ( e ) Raw traces showing that ghrelin did not change the firing rate of the example neuron in Tg mice. ( f ) In Tg mice, the firing rate of neurons (8/11) was not increased in the presence of 100 nM ghrelin (n.s. ghrelin versus control, t =1.112, Paired t -test). ( g ) Statistical analysis of d and f . Each bar represents the mean±s.e.m. Full size image Enhanced dopamine turnover and release by ghrelin The data from brain slice recordings revealed that ghrelin increased spontaneous activity of dopaminergic neurons. To investigate the effect of ghrelin on dopamine release, we determined the rate of in vitro dopamine turnover using high-performance liquid chromatography (HPLC). Adult female Wistar rats weighing 200~250 g were divided into four groups. Dopamine content and its metabolites, DOPAC and HVA, in striatum were detected, and the turnover rate was calculated as the combination of DOPAC and HVA versus dopamine. The results showed that both DOPAC and HVA levels were elevated after intracerebroventricular (i.c.v) injection of 100 nM or 1,000 nM ghrelin (5 μl), and the turnover rate was also increased ( Fig. 7a–d ), suggesting that ghrelin increased dopamine release. To confirm this result, carbon fibre electrodes were placed in the striatum for detecting dopamine release by electrical stimulation of medial forebrain bundles. i.c.v. injection of ghrelin (1,000 nM, 5 μl) caused nearly a threefold increase of dopamine release from 1.3±0.2 μM to 3.9±0.5 μM ( n =6, P <0.01) in the striatum ( Fig. 7e ), confirming the increased release and turnover rate of dopamine by ghrelin. 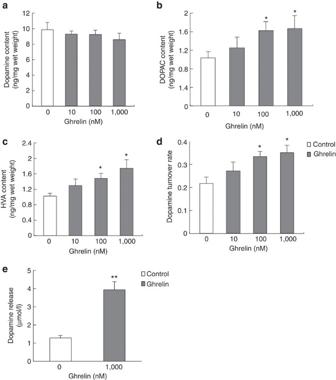Figure 7: i.c.v injection of ghrelin increases dopamine release and turnover rate in the striatum. (a–d) Contents of dopamine and its metabolites in rat striatum were measured using HPLC. (a) Striatal dopamine levels of groups before and after i.c.v. injections of ghrelin (10–1,000 nM, in 5 μl).n=6. Each bar represents the mean±s.e.m. (b) Striatal DOPAC levels were increased after treatment with 100 and 1,000 nM ghrelin (n=6. Each bar represents the mean±s.e.m. *P<0.05, Ghrelin versus Control). (c) Striatal HVA levels were increased after treatment with 100 and 1,000 nM ghrelin (n=6. Each bar represents the mean±s.e.m. *P<0.05, Ghrelin versus Control). (d) i.c.v. injection of ghrelin (100 and 1,000 nM) increased the dopamine turnover rate (n=6. Each bar represents the mean±s.e.m. *P<0.05, Ghrelin versus Control). (e) Dopamine releasein vivoevoked by stimulation of the medial forebrain bundles was recorded with carbon fibre electrodes in the striatum using fast cyclic voltammetry. Ghrelin (i.c.v. 1,000 nM, 5 μl) significantly increased the dopamine release from 1.3 ±0.2 μM to 3.9±0.5 μM (n=6. Each bar represents the mean±s.e.m. **P<0.01, Ghrelin versus Control). Figure 7: i.c.v injection of ghrelin increases dopamine release and turnover rate in the striatum. ( a – d ) Contents of dopamine and its metabolites in rat striatum were measured using HPLC. ( a ) Striatal dopamine levels of groups before and after i.c.v. injections of ghrelin (10–1,000 nM, in 5 μl). n =6. Each bar represents the mean±s.e.m. ( b ) Striatal DOPAC levels were increased after treatment with 100 and 1,000 nM ghrelin ( n =6. Each bar represents the mean±s.e.m. * P <0.05, Ghrelin versus Control). ( c ) Striatal HVA levels were increased after treatment with 100 and 1,000 nM ghrelin ( n =6. Each bar represents the mean±s.e.m. * P <0.05, Ghrelin versus Control). ( d ) i.c.v. injection of ghrelin (100 and 1,000 nM) increased the dopamine turnover rate ( n =6. Each bar represents the mean±s.e.m. * P <0.05, Ghrelin versus Control). ( e ) Dopamine release in vivo evoked by stimulation of the medial forebrain bundles was recorded with carbon fibre electrodes in the striatum using fast cyclic voltammetry. Ghrelin (i.c.v. 1,000 nM, 5 μl) significantly increased the dopamine release from 1.3 ±0.2 μM to 3.9±0.5 μM ( n =6. Each bar represents the mean±s.e.m. ** P <0.01, Ghrelin versus Control). Full size image Ghrelin-KCNQ pathway attenuates haloperidol-induced catalepsy To test the in vivo effect of ghrelin, we utilized the rat model of catalepsy induced by haloperidol, a specific D2 receptor antagonist that causes symptoms of PD. The administration of haloperidol (5 mg kg −1 , intraperitoneal (i.p.)) induced symptoms of catalepsy with characteristics of rigidity and akynesia posturing that lasted for more than 1 h. As a control, unilateral microinjection of saline (0.5 μl) into SNc did not produce a posturing behaviour in catalepsy rats ( Fig. 8a ). In contrast, unilateral injection of ghrelin (1,000 nM in 0.5 μl) into SNc induced a significant contralateral dystonic posturing ( Fig. 8a ). 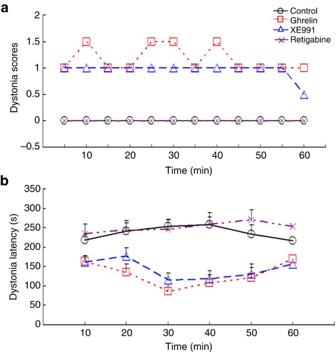Figure 8: Ghrelin attenuates haloperidol-induced catalepsyin vivo. (a) Effects of ghrelin on postural behaviour in rats receiving systemic administration of haloperidol. The line graph shows the scores of deviated posturing in rats recorded in 60 min after microinjection of ghrelin (1,000 nM, 0.5 μl), XE991 (1 μM, 0.5 μl) or retigabine (5 μM, 0.5 μl) into the SNc. (b) Time course of the bar tests shows that microinjection of ghrelin or XE991 into the SNc significantly attenuated the descent latency time in haloperidol-induced catalepsy rats (n=7. Each bar represents the mean±s.e.m. **P<0.01, Ghrelin versus Control; XE991 versus Control; non-parametric one-way Kruskal–Wallis test followed by the Mann–Whitney test). The deviated posturing appeared immediately and persisted for at least 1 h. Figure 8: Ghrelin attenuates haloperidol-induced catalepsy in vivo . ( a ) Effects of ghrelin on postural behaviour in rats receiving systemic administration of haloperidol. The line graph shows the scores of deviated posturing in rats recorded in 60 min after microinjection of ghrelin (1,000 nM, 0.5 μl), XE991 (1 μM, 0.5 μl) or retigabine (5 μM, 0.5 μl) into the SNc. ( b ) Time course of the bar tests shows that microinjection of ghrelin or XE991 into the SNc significantly attenuated the descent latency time in haloperidol-induced catalepsy rats ( n =7. Each bar represents the mean±s.e.m. ** P <0.01, Ghrelin versus Control; XE991 versus Control; non-parametric one-way Kruskal–Wallis test followed by the Mann–Whitney test). Full size image Bar test is another established assay that is used for measuring haloperidol-induced catalepsy. A total of 14 rats (7 in each group) were injected intraperitoneally with haloperidol (0.5 mg kg −1 ). Injection of ghrelin (1,000 nM) in 0.5 μl into SNc resulted in shortening of descent latency ( Fig. 8b ). In haloperidol-treated group, the descent latency of bar test was from 257.7±19.1 s to 216.9±24.7 s ( n =7). Local microinjection of ghrelin (1,000 nM) significantly reversed the haloperidol-induced catalepsy ( n =7, P <0.01). The anticataleptic effect was significant from 20 to 40 min with the peak appearing at 30 min (86±24.6 s versus 252.6±15.6 s) ( Fig. 8b ). Administration of XE991 (1 μM, 0.5 μl) into the SNc mimicked the anticataleptic effects of ghrelin in postural and bar tests, whereas KCNQ channel opener retigabine (5 μM, 0.5 μl) had no effect ( Fig. 8 ). In contrast, co-application of retigabine and ghrelin antagonized the effect of ghrelin on catalepsy ( Supplementary Fig. S3 ). These results suggest that activation of ghrelin-KCNQ pathway in SNc can attenuate the haloperidol-induced catalepsy in vivo . In this study, as summarized in Supplementary Fig. S4 , our findings reveal a novel mechanism by which ghrelin enhances dopaminergic neuronal firing by inhibiting native KCNQ/M-current through GHS-R-PLC-PKC pathway. The enhanced excitability induced by ghrelin results in accelerated release and turnover of dopamine in the striatum, and attenuation of catalepsy elicited by systemic haloperidol administration in vivo . Previous investigations show that ghrelin stimulates release of neurotransmitters [11] , and induces depolarization by inhibiting K + conductance [29] . To identify the downstream effector for ghrelin-mediated effect on excitability of nigral dopaminerigc neurons, we hypothesized that ghrelin might affect neuronal Kv7/KCNQ/M-channels that are predominantly expressed in the CNS and have a profound effect on membrane excitability [32] , [33] . This hypothesis was based on observations that the pathway activated by binding of ghrelin to its G-protein-coupled receptor GHS-R1a regulates the activation of downstream PLC that depletes membrane PIP 2 levels [13] and activates PKC. The depletion of PIP 2 or phosphorylation of KCNQ channels by PKC can lead to a suppression of neuronal voltage-gated Kv7/KCNQ/M-channel activity [24] . In addition, KCNQ2 immunoactivity is also found somatically in SNc [15] . All these studies suggest that ghrelin signalling is likely coupled with Kv7/KCNQ channel function. To demonstrate the effect of ghrelin on native KCNQ/M-current in nigral dopaminergic neurons that is extremely small, we performed nystatin-perforated patch clamp recordings. The typical KCNQ/M-current recorded in nigral dopaminergic neurons from brain slices is less than 50 pA with characteristic deactivation kinetics when stepped from −20 mV (for opening KCNQ/M-current) to −40 mV (for deactivation of KCNQ/M-current). The KCNQ/M-current deactivation kinetics features KCNQ2 channels that have been shown to be expressed in nigral dopaminergic neurons [15] , [18] . In addition, although previous studies have shown that the signal transduction pathway for ghrelin is mediated by PLC/PKC in non-neuronal tissues and cell lines [13] , [27] , [28] , our findings first demonstrated that PKC is involved in the effects of ghrelin in native neurons. The signalling transduction pathway of how ghrelin promotes nigral neuronal firing is summarized in Supplementary Fig. S4 . Binding of ghrelin to its receptor GHS-R1a causes the activation of PLC and the following hydrolyzation of PIP 2 . The product of PIP 2 hydrolyzation, diacylglycerol (DAG), activates PKC, resulting in the phosphorylation of KCNQ channels (for example, S541 of KCNQ2) [34] and its closure, which elicits reduced outward potassium current and enhances neuronal excitability of SNc dopamine neurons. To further confirm the role of ghrelin/KCNQ pathway in regulating neuronal excitability, we chose DRG neurons and CA1 hippocampal pyramidal neurons where the expression of both ghrelin receptors and KCNQ channels are robust, and KCNQ channels have profound effects on neuronal excitability [10] , [17] , [35] , [36] . The KCNQ/M-currents in small DRG neurons are large with less contamination of other currents, and therefore are more reliable and suitable for pharmacological manipulations [17] , [37] . Because DRG neurons are highly refractory to fire repetitively, another characteristic of KCNQ-expressing neurons, we utilized a higher concentration of ghrelin (300 nM) in this study. To further demonstrate the ghrelin signalling-KCNQ pathway, we took advantage of Tg mice expressing a dominant negative KCNQ2 pore mutation that causes repetitive neuronal firing [31] , [38] . Our findings show that ghrelin increases firing frequency of CA1 neurons from WT mice that normally are silent or fire slowly [38] , [39] , but fails to modulate the firing of CA1 neurons from Tg mice where native KCNQ/M-current is suppressed. This indicates that ghrelin serves as an upstream signalling molecule and enhances neuronal spiking through inhibition of Kv7/KCNQ channels. Most interestingly, ghrelin is able to modulate native Kv7/KCNQ channels expressed in nigral dopaminergic neurons, small DRG neurons and CA1 pyramidal neurons. In addition to the indicated three different types of neurons, ghrelin receptor and Kv7/KCNQ channels are also individually expressed in pituitary, neuropeptide Y neurons in hypothalamus and cortex [21] , [40] , [41] , [42] , all of these suggest that the ghrelin signalling and Kv7/KCNQ suppression are likely common pathways primarily utilized by the central nervous system. Neuronal excitability is closely linked to dopamine release in the brain [43] and increased firing of dopamine neurons accelerates the dopamine release in the striatum, nucleus accumbens and cerebral cortex [43] , [44] . The present study shows that ghrelin increases firing rate dose dependently, and results in the burst firing at high concentrations. To demonstrate the in vivo effect of ghrelin, we utilized the catalepsy model induced by a specific D2 receptor antagonist haloperidol, which has been proven to represent a reliable model for PD and is selectively reversed by clinically effective antiparkinson drugs [45] . Based on the current understanding of neural framework in basal ganglia, degeneration of nigral dopaminergic neurons leads to dopamine depletion in the striatum, resulting in an imbalance of direct and indirect pathway and subsequent motor disorders [46] , [47] , [48] . Unilateral microinjection of ghrelin causes the contralateral posturing and anticatalepsy effect, which is likely resulted from enhanced dopamine release induced by ghrelin directly and further activates the pathway of basal ganglia from the ipsilateral cortex. This was further confirmed by our in vitro and in vivo studies that intracerebroventricular injection of ghrelin in rats produces a dramatic enhancement of dopamine turnover rate and dopamine release in the striatum, which is in accordance with the studies that intraperitoneal administration of ghrelin improves the impairment of rota-rod performance in mouse MPTP-induced PD models [49] by stimulating dopamine overflow or dopamine turnover in the nucleus accumbens [9] , [12] , [50] , [51] . All together, our findings show that ghrelin, via specific blockage of KCNQ channel function, can increase the firing of mesencephalic dopaminergic neurons and mediate anticataleptic effects. Therefore, ghrelin signalling and ghrelin-mediated inhibition of Kv7/KCNQ/M-current might provide therapeutic potential for alleviation of PD symptoms. Animals and chemical reagents Animals (Sprague-Dawley (SD) rats of postnatal 7 days and 10 days, 6- to 7-week-old rQ2-G279S Tg mice with background of TB6D2F1/Crl × C57/B6, adult Wistar rats) were housed (two to five per cage for adult animals) under a controlled temperature (23±2 °C) and humidity (50±5%) environment with ad libitum access to food and water, and kept in a 12-h light/dark cycle. All procedures were carried out in accordance with the guidelines of the Animal Ethics Committee of Qingdao University and Peking University. Cell culture reagents were from Gibco (Grand Island, NY, USA). Ghrelin (Tocris Bioscience) was dissolved in water into 10 −4 M, and XE991 (Tocris Bioscience) was dissolved in dimethylsulphoxide (DMSO) into 40 mM. All solutions were stored at −80 °C and diluted on the day of use. Other chemicals and regents used were from Sigma. Brain slice preparation Brain slices of the SNc were prepared from SD rats of postnatal 10 days. Brains were rapidly removed and immersed in ice-cold oxygenated (95% O 2 /5% CO 2 ) cutting solution containing (in mM): 110 choline chloride, 2.5 KCl, 0.5 CaCl 2 , 7 MgCl 2 ·6H 2 O, 1.3 NaH 2 PO 4 , 25 NaHCO 3 , 25 glucose, 1.3 Na L -ascorbate, 0.6 Na-pyruvate. Coronal slices (300 μm) containing SNc were cut on a vibratome (Leica VT1000S), then incubated in oxygenated artificial cerebrospinal fluid (in mM: 125 NaCl, 2.5 KCl, 1.3 NaH 2 PO 4 , 1.3 MgCl 2 ·6H 2 O, 2 CaCl 2 , 25 NaHCO 3 , 10 glucose, 1.3 Na L -ascorbate, 0.6 Na-pyruvate), and allowed to recover for 1 h at 34 °C before experiment. For experiments with recordings of hippocampal brain slices, Tg mice (rQ2-G279S) were used [31] . The transverse hippocampal slices were prepared according to procedure previously reported [52] , and the solutions used were the same as rat brain slices. Whole-cell patch clamp recordings After equilibration, brain slices were transferred to a small volume chamber (~0.5 ml) that was mounted on an upright fixed stage of Infra-Red Differential Interference Contrast microscope (Nikon, Japan). The chamber was superfused with oxygenated artificial cerebrospinal fluid at a flow rate of 1.5~2.0 ml min −1 at room temperature (22–25 °C). Patch pipettes with resistance of 2~4 MΩ were pulled from borosilicate glass capillaries with a horizontal puller (P-97, Sutter Instrument, Novato, CA, USA). The internal solution (290 mOsm) contained (in mM) 130 K-gluconate, 10 HEPES, 0.6 EGTA, 5 KCl, 4 MgCl 2 ·6H 2 O, 3 Na 2 ATP, 0.3 Na 3 GTP and 10 Na 2 -phosphocreatine, pH 7.3 with KOH. Whole-cell patch clamp recording of SNc neurons was carried out to record spikes under current-clamp mode using a Multiclamp 700B amplifier (Molecular Devices, Union City, CA). Electrophysiological data were acquired at 5 or 10 kHz with a Digital 1440A interface (Molecular Devices) in conjunction with a PC and were analysed by pClamp10 (Molecular Devices). Nystatin-perforated patch clamp recordings Nystatin-perforated patch clamp technique was employed to record native KCNQ/M-current in SNc and hippocampus. The internal solution (290 mOsm) containing (in mM) 60 K-acetate, 60 KCl, 1 CaCl 2 , 2 MgCl 2 , 40 HEPES, pH 7.2 adjusted with KOH. Nystatin (Sigma, 0.5 mg ml −1 in DMSO) was freshly made just before recording. The nystatin solution was added into internal solution to a final concentration of 200 μg ml −1 , and the electrode was backfilled with the internal solution. Primary cultures of DRG neurons and whole-cell patch clamp recordings DRG neurons were dissected from 7-day-old SD rats and prepared using an enzymatic dissociation procedure. Briefly, DRGs from all spinal levels were dissected aseptically and collected in DMEM medium supplemented with 10% fetal bovine serum (FBS). After washing twice with cold PBS, DRG neurons were incubated for 45 min at 37 °C in 3 mg ml −1 collagenase, and then incubated for further 10 min in 0.25% trypsin. Ganglia were then mechanically triturated with a fire-polished glass Pasteur pipette, centrifuged and re-suspended in DMEM medium supplemented with 10% FBS and 100 U penicillin/streptomycin. Cells were incubated at 37 °C for 4 h to allow cells to adhere to the substrate and then changed to the neurobasal medium supplemented with 2% FBS, 2% horse serum, 1% B27 and 1% L -glutamine. For recordings, dissociated neurons were plated onto plastic dishes coated with poly- L -lysine and used 3–8 days in culture. The external solution contained (in mM): 144 NaCl, 2.5 KCl, 0.5 MgCl 2 ·6H 2 O, 2 CaCl 2 , 5 HEPES and 10 glucose, pH 7.4 adjusted with NaOH. Pipettes were filled with intracellular solution containing (in mM): 140 KCl, 2 MgCl 2 ·6H 2 O, 0.14 CaCl 2 , 4 EGTA, 10 HEPES, pH 7.2 adjusted with KOH. Immunostaining of GHS-R1a The Tg mice were transcardially perfused with saline followed by 4% paraformaldehyde in 0.1 M PBS buffer, pH 7.4. The brains were removed and then immersed in the fixative at 4 °C for 16 h. Then the brains were transferred to 20% sucrose in 0.1 M PBS for 48 h. Twenty-micrometer serial coronal sections were cut. The sections were first rinsed in 0.01 M PBS for 3 × 10 min, in 0.01 M PBS with 0.3% Triton X-100 (TX; Sigma-Aldrich, St Louis, MO) for 30 min, 10% normal goat serum to block nonspecific binding sites. Then they were incubated with antibody against GHS-R1a (1:1,000) (Phoenix Pharmaceuticals, Brulingame, CA) in a 0.01 M PBS buffer containing 0.3% Triton X-100 and 10% normal goat serum at 4 °C for 36 h. After rinsing with PBS, the sections were incubated with secondary Alexa Fluo 555 anti-rabbit IgG (1:500) in a 0.01 M PBS buffer containing 0.3% Triton X-100 at room temperature for 2 h. Finally, the sections were rinsed in 0.01 M PBS and mounted with glycerol. Immunofluorescence was analysed using confocal microscopy. HPLC electrochemical detection (HPLC-ECD) Adult female Wistar rats weighing 200~250 g were anesthetized with chloral hydrate (400 mg kg −1 , i.p.). Ghrelin or saline in 5 μl was microinjected into the cerebral ventricle using stereotaxic techniques. Rats in different experimental groups were killed 3 h after ghrelin or saline injection. Both sides of striatum were carefully isolated and transferred to liquid nitrogen for storage. The levels of the striatal dopamine and its metabolites, DOPAC and HVA, were determined with HPLC equipped with a 2465 electrochemical detector (Waters Corp, Milford, Massachusetts, USA) as described previously [53] , [54] , [55] . Data were presented as ng mg −1 wet weight of brain tissue. Fast cyclic voltammetry Adult female Wistar rats were anesthetized with chloral hydrate (400 mg kg −1 , i.p.). Dopamine release in the striatum evoked by electrical stimulation of the medial forebrain bundles 3 h after ghrelin or saline injection into cerebral ventricle was determined by fast cyclic voltammetry as previously reported [54] , [55] , [56] , [57] . Following each experiment in vivo , the working electrode was calibrated in vitro in standard dopamine solutions (0.01~5.00 μM). Histological examinations of brain slices were adopted to ensure that the positions of stimulating electrode and working electrode were accurate. Postural test and bar test Adult female Wistar rats weighing 200~250 g were anesthetized and placed in a stereotaxic frame. A guide cannula (outer diameter: 0.4 mm; inner diameter: 0.3 mm) was implanted into the left SNc using stereotaxic techniques (AP: −5.6 mm, ML: 1.6 mm, V: −8 mm). The cannula was then anchored to the skull with stainless steel screws and dental acrylic. Stainless steel stylets were used to keep the cannula sealed and prevent occlusion. Rats were placed in an observation cage to which they had already become habituated after recovery. All behavioural tests were performed during 12:00~17:00 to minimize the influence of circadian rhythm. To induce catalepsy, rats were injected with haloperidol (5 mg kg −1 , i.p.). A stainless-steel injector needle inserted inside the implanted guide cannulas was connected via a polyethylene catheter to Hamilton micro syringes (1 μl). At 60 min after haloperidol administration, solution of saline or ghrelin (1,000 nM) in 0.5 μl was microinjected into the SNc over a 2-min period. At the end of injection, the injection cannula was kept in SNc for an additional 1 min before removal and then replaced by a stylet. According to the angle between the nose-back line and back-tail line of rats, the postural asymmetry was quantitatively scored as follows: 0, no fixed postural alteration; 1, less than 30°; 2, 30~59°; 3, 60~89°; 4, 90° and greater [58] , [59] . Bar test (a horizontal, cylindrical metal bar, diameter 1 cm, height 9 cm above the floor) was carried out to assess catalepsy (rigidity and akinesia). At 60 min after haloperidol administration, saline or ghrelin (1,000 nM) in 0.5 μl was microinjected into the SNc over a 2-min period. Both forepaws of rats were placed on the bar. The degree of catalepsy was assessed by measuring the time from placement of rats until removal of one of its paws (‘descent latency’) with a cutoff time of 300 s (ref. 45 ). Statistical analysis All data were presented as mean±s.e.m. Differences between means in two groups were compared using the paired or unpaired t -test, and one-way analysis of variance followed by the Student-Newman-Keuls test was used to compare difference for more than two groups. The data for HPLC were analysed by the Rank–Sum test. The scores of deviated posturing and the total time spent by rats in bar tests were analysed by the non-parametric one-way Kruskal–Wallis test followed by the Mann–Whitney test. P -value less than 5% was considered to be statistically significant. How to cite this article: Shi, L. et al. Peptide hormone ghrelin enhances neuronal excitability by inhibition of Kv7/KCNQ channels. Nat. Commun. 4:1435 doi: 10.1038/ncomms2439 (2013).